Magnetic and electric coherence in forward- and back-scattered electromagnetic waves by a single dielectric subwavelength sphere Magnetodielectric small spheres present unusual electromagnetic scattering features, theoretically predicted a few decades ago. However, achieving such behaviour has remained elusive, due to the non-magnetic character of natural optical materials or the difficulty in obtaining low-loss highly permeable magnetic materials in the gigahertz regime. Here we present unambiguous experimental evidence that a single low-loss dielectric subwavelength sphere of moderate refractive index ( n =4 like some semiconductors at near-infrared) radiates fields identical to those from equal amplitude crossed electric and magnetic dipoles, and indistinguishable from those of ideal magnetodielectric spheres. The measured scattering radiation patterns and degree of linear polarization (3–9 GHz/33–100 mm range) show that, by appropriately tuning the a/λ ratio, zero-backward (‘Huygens’ source) or almost zero-forward (‘Huygens’ reflector) radiated power can be obtained. These Kerker scattering conditions only depend on a/λ . Our results open new technological challenges from nano- and micro-photonics to science and engineering of antennas, metamaterials and electromagnetic devices. Electromagnetic scattering by small particles compared with the wavelength is a topic of great interest to fields extending from telecommunications, astrophysics or meteorology to biophysics and material science [1] , [2] , [3] . The increasing demand of wireless device miniaturization for communication and sensor applications, and the search of new materials with electromagnetic properties ‘à la carte’, has fostered a renewed interest in subwavelength particles as basic building blocks for controlling optical radiation at subwavelength scales. These issues underline the emerging concepts of metamaterial inspired microwave and radio-wave electrically small antennas [4] and their optical analogues, either dielectric [5] , [6] or based on plasmon subwavelength optics [7] . A key ingredient for relevant applications involves an optimal design of the electric and magnetic responses to the incident electromagnetic wave in small structures of lossless magnetodielectric materials. Hypothetical particles exhibiting both electric and magnetic dipolar resonances scatter with coherent effects between both dipoles, hence their use enables control of the scattered radiation, as predicted long ago by Kerker et al . [8] ; that is, under certain conditions for the values of the electric permittivity ε and magnetic permeability μ (known as ‘Kerker conditions’), the response of a particle to plane-wave illumination consists of equal amplitude crossed electric- and magnetic-induced dipoles. When they oscillate in-phase, the scattered fields are mainly in the direction of the incoming wave, with zero-backward radiated power, (‘first Kerker’ or ‘zero-backward intensity condition’) and correspond to an ideal ‘Huygens’ secondary source [9] . Such sources are interesting as elements of electrically small antennas [10] , [11] . Correspondingly, at the ‘second Kerker condition’ (or ‘near-zero-forward intensity condition’) the dipoles are out-of-phase, (‘Huygens reflector’), which opens intriguing applications for metamaterials and cloaking [12] . However, achieving such magnetodielectric behaviour has been prevented because of the absence of natural magnetic media at optical frequencies and to the lossy magnetic materials in the microwave regime. Recent reports on the observation of zero-forward scattering by magnetic spheres [13] , [14] according to Kerker criteria [8] was questioned [15] , [16] , [17] . Thus to date there has been no unambiguous experimental evidence. The large losses in metallic structures and metamaterials have turned attention to high-permittivity subwavelength low-loss particles with non-overlapping magnetic or electric dipolar resonances [18] , [19] , [20] , [21] , [22] , [23] . In particular, dielectric subwavelength spheres of moderate permittivity like silicon [24] , [25] present strong magnetic and electric dipolar resonances in the visible, as well as in telecom and near-infrared frequencies, where silicon absorption is negligible, without spectral overlap between quadrupolar and higher-order modes [25] . Similar effects are expected for other semiconductor materials [25] , [26] like germanium ( ε ≈16 in the infrared) and rutile-TiO 2 with an effective permittivity as low as ε ≈6 in the near-infrared. The observation of the strong magnetic response predicted in silicon nanoparticles has recently been reported [27] . Interestingly, the spectral proximity between dipolar electric and magnetic responses allows coherent effects between them. In particular, when the absolute values of electric and magnetic polarizabilities are the same, such non-magnetic particles present differential scattering cross-sections [26] equivalent to those predicted for hypothetical dipolar magnetodielectric particles [8] . Dielectric spheres are fully scalable with identical properties from DC to light. The ratio λ/ ( na ) constitutes a scaling factor that keeps the effects in the angular distribution of scattered intensity derived from the aforementioned interference between the induced electric and magnetic dipoles, (this magnetodielectric behaviour was actually proven for dielectric cylinders, rescaled from those being made of ceramic in the microwave region to those of Si in the near-infrared [28] ). Here we use the same argument for spheres: the similar value of λ /( na ) in the experiments carried out in this paper should be compared with that of a Si sphere in the near-infrared [25] , [26] . Control over the angular distribution of scattered radiation by using subwavelength dielectric elements will then be an important step in nano and mesoscopic photonic sciences. Their low absorption minimizes thermal heating and absorption losses, as well as those of the CMOS integration of current plasmonic devices [29] . At the same time, they strongly reduce the vulnerability of radiofrequency communication systems to high-power electromagnetic pulses [22] . Concerning spheres, for a given refractive index n and working wavelength λ , it will be possible to select the ‘Huygens’ source or reflector mode by choosing the appropriate sphere radius a (ref. 26 ). An all-dielectric Yagi-Uda antenna based on these ideas was recently proposed [6] , [30] and experimentally tested in the microwave regime [31] . The scattering anisotropy also has a key role in the mechanical action of electromagnetic fields on small particles. The radiation pressure, which until now was believed to push objects [32] , [33] , has recently been designed to exert a pulling action towards the source, as recently proposed on exciting the induced magnetic dipole or multipoles of the particle [34] , [35] , and by appropriately designing the illuminating wave-field angular spectrum [36] . Here we study the electromagnetic scattering from a single isotropic homogeneous dielectric subwavelength sphere of radius a made of moderately high-refractive index ( n ≈3–4) under plane-wave illumination. This is the simplest, textbook-like, example of particle radiating fields identical to those from crossed electric and magnetic dipoles. It is remarkable that this basic example of ‘anomalous’ scattering, concerning the anisotropy of the polarization of radiated fields, has not yet been experimentally realized. By measuring the angular radiation pattern of microwave scattering from this single subwavelength sphere, we provide experimental evidence of both zero-backward and near-zero-forward scattering, at specific a/λ ratios. Also, polarization of the scattered radiation contains worthy complementary information. Our measurements of the degree of linear polarization of the scattered radiation [1] , [2] are in full agreement with the behaviour predicted for magnetodielectric particles [37] , [38] . From a fundamental point of view, our results represent the first experimental confirmation of Kerker’s proposal concerning unconventional forward–backward scattering asymmetry from a single subwavelength sphere. Scattering by a subwavelength dielectric sphere The field scattered by a homogeneous dielectric sphere illuminated by a plane wave can be decomposed into a multipole series (the so-called Mie expansion), characterized by the electric and magnetic Mie coefficients { a n } and { b n }, respectively; ( a 1 and b 1 being proportional to the electric and magnetic dipoles, a 2 and b 2 to the quadrupoles, and so on) [1] . For very-long wavelengths ( a / λ <<1) the scattered field is dominated by a small electric dipolar response ( a 1 ); however, as the wavelength decreases the first spectral resonance always corresponds to a magnetic dipolar term ( b 1 ). The scattering phenomena predicted in the near-infrared for semiconductors nanospheres [26] , and in particular the electroinductive and magnetoinductive eigenmodes, have their origin in the spectral overlap between the first (magnetic) and second (electric) ‘Mie’ resonances. These are reminiscences of electric and magnetic whispering gallery modes. On resorting to the theory on magnetodielectric spheres reported in our previous work [25] , [26] , [39] , and that on Si and ceramic cylinders [28] , and recalling the scaling ratio λ /( na ) that maintains the existence of these phenomena in different frequency ranges, we also predict similar observations in conventional semiconductor spheres in the near-infrared. The rescaling property of our scattering problem, together with the intrinsic interest that our results have in technological applications in the microwave range (electrically small antennas) aimed us to perform our simulations and experiments in the microwave regime ( v ~3–9 GHz→ λ ~33–100 mm) [15] . A millimetre spherical dielectric particle of radius a =9 mm with moderately high electric permittivity ε ≈16 should be expected to have magnetodielectric scattering effects and thus angular-scattered intensity distributions similar to those recently predicted in the near-infrared [26] for semiconductor nanospheres. The predicted results for either Si or Ge nanospheres of 240 nm radius in the near-infrared ( ε ≈16 for λ ~1.2–2.4 μ m) can be rescaled to our millimetre size spheres with 9 mm in the gigahertz regime ( ε ≈16 for λ ~33–100 mm) with the same radius to wavelength ratio ( a/λ ~0.1–0.2). The experimental setup and experimental details are shown in Fig. 1 , Methods, and Supplementary Methods . 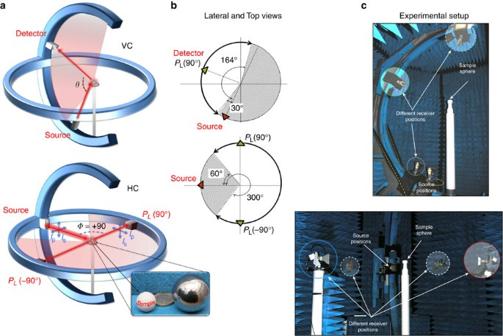Figure 1: Experimental microwave setup. (a) 3D schematics of the two scattering configurations (vertical (VC) in the top and horizontal (HC) in the bottom) designed to measure the scattering patterns and the linear polarization degree, respectively, of a single subwavelength spherical scatterer of radiusa=9 mm andε=16.5+0i(provided by Emerson and Cuming (http://www.eccosorb.eu/)). The sample (white sphere shown in the inset) is illuminated and analysed using parallel (p) and perpendicular (s) polarizations to the scattering plane (pink areas). (b) Lateral and top views respectively of the VC and HC configurations, depicting the experimentally accessed angular range. (c) Photographs of the real experimental setup arranged in VC (top) and HC (bottom) configurations, and fully embedded in an anechoic chamber. Figure 1: Experimental microwave setup. ( a ) 3D schematics of the two scattering configurations (vertical (VC) in the top and horizontal (HC) in the bottom) designed to measure the scattering patterns and the linear polarization degree, respectively, of a single subwavelength spherical scatterer of radius a =9 mm and ε =16.5+0 i (provided by Emerson and Cuming ( http://www.eccosorb.eu/ )). The sample (white sphere shown in the inset) is illuminated and analysed using parallel (p) and perpendicular (s) polarizations to the scattering plane (pink areas). ( b ) Lateral and top views respectively of the VC and HC configurations, depicting the experimentally accessed angular range. ( c ) Photographs of the real experimental setup arranged in VC (top) and HC (bottom) configurations, and fully embedded in an anechoic chamber. 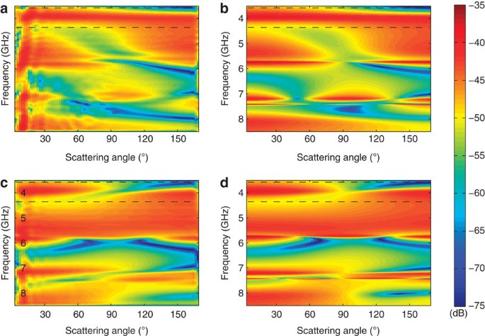Figure 2: Scattered intensity by a subwavelength dielectric sphere. Colour map of the magnitude (in dB) of the scattered field, both experimental (a) and simulated (b), of the studied target (sphere of radiusa=9 mm andε=16.5+0i,μ=1) as a function of the incident frequency (vertical axis in GHz) and the scattering angle (horizontal axis in degrees from 0° (forward) to 180° (backward)) when the incident beam is linearly polarized parallel to the scattering plane (p polarization). If the incident polarization is perperdicular to the scattering plane (s polarization), the magnitude of the scattered intensity, both experimental and simulated, are displayed in (c) and (d), respectively. Black dashed lines mark the incident frequencies for which Kerker conditions hold in the dipolar regime: upper line corresponds to the zero-backward condition (first Kerker condition) and bottom one to the zero-forward condition (second Kerker condition)8. Full size image Figure 2 summarizes our experimental results in a colour map of the magnitude (in dB) of the scattered field of the target as a function of the incident frequency (in GHz) and the scattering angle (in degrees) when the incident beam is linearly polarized parallel (p) or perpendicular (s) to the scattering plane, respectively. The simulated results computed according to Mie theory for the considered spherical target are also shown, with an amazing overall agreement with the experiments. In order to get some insight into these results, in Fig. 3a , we show the spectral evolution of the normalized extinction cross-section (black solid line) calculated according to Mie theory for the considered spherical target ( ε ≈16.5+0 i ) [1] . In order to facilitate the identification of the different multipolar contributions, the first four multipolar terms of the normalized scattering cross-section Q ext =σ ext /a 2 , corresponding to dipolar and quadrupolar contributions, both electric and magnetic, are also plotted [1] . These are directly associated with Mie coefficients a 1 , a 2 , b 1 and b 2 . From the spectral profile of Q ext and their dipolar contributions, both an electroinductive and a magnetoinductive resonance at λ= 57 and λ= 76 mm can be identified, respectively (quadrupolar terms a 2 , b 2 present resonant modes for incident wavelengths around 42 and 52 mm, respectively). In the dipolar region (grey area in Fig. 3a ), where the scattering is perfectly described by a 1 and b 1 , it is easy to show that the theoretical differential scattering cross-section in the scattering plane is simply given by (see Methods) Figure 2: Scattered intensity by a subwavelength dielectric sphere. Colour map of the magnitude (in dB) of the scattered field, both experimental ( a ) and simulated ( b ), of the studied target (sphere of radius a =9 mm and ε =16.5+0 i , μ =1) as a function of the incident frequency (vertical axis in GHz) and the scattering angle (horizontal axis in degrees from 0° (forward) to 180° (backward)) when the incident beam is linearly polarized parallel to the scattering plane (p polarization). If the incident polarization is perperdicular to the scattering plane (s polarization), the magnitude of the scattered intensity, both experimental and simulated, are displayed in ( c ) and ( d ), respectively. Black dashed lines mark the incident frequencies for which Kerker conditions hold in the dipolar regime: upper line corresponds to the zero-backward condition (first Kerker condition) and bottom one to the zero-forward condition (second Kerker condition) [8] . 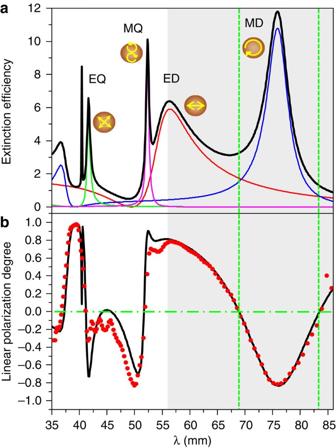Figure 3: Extinction efficiency and linear polarization degree at the right-angle scattering configurationPL(90°). (a) Mie calculations of the extinction efficiency (Qext) as a function of the incident wavelengthλ(in mm) of a dielectric subwavelength sphere (a=9 mm,ε=16.5+0i). The totalQext(black solid line) and their first four multipolar contributions: electric dipolar (red), magnetic dipolar (blue), electric quadrupolar (green) and magnetic quadrupolar (pink) are included. The grey area corresponds to the spectral range where dipolar terms dominate. In this region,Qextpresents two main peaks due to the excitation of either an electric dipolar (ED atλ=57 mm) or a magnetic dipolar (MD atλ=76 mm) resonance. Higher-order resonances are also observed (EQ: electric quadrupolar, MQ: magnetic quadrupolar). These resonant modes are consequence of the distribution of the electric field inside the particle (see inset which symbolically represents this distribution). (b) In the dipolar regime (grey area), the linear polarization degree at the right angle configuration,PL(90°), also identifies dipole resonances: the electric (positive values) and the magnetic (negative values). Experimental values ofPL(90°) for the considered target (a=9 mm andε=16.5+0i) averaged over the different experimental configurations described inFig. 1(VC and +90° and –90° for the HC) are plotted as red dots. In addition, theoretical values ofPL(90°) (see equation 5) are also included (black solid line) to show the excellent agreement between theory and experiment, even out of the dipolar regime (λ<53 mm). Horizontal dot-dashed line corresponds toPL(90°)=0. Dotted vertical lines mark the incident wavelengths at which dipolar contributions, either electric or magnetic, cross each other (a). These wavelengths also coincide with those at whichPL(90°)=0 (b). Full size image Figure 3: Extinction efficiency and linear polarization degree at the right-angle scattering configuration P L (90°). ( a ) Mie calculations of the extinction efficiency ( Q ext ) as a function of the incident wavelength λ (in mm) of a dielectric subwavelength sphere ( a =9 mm, ε =16.5+0 i ). The total Q ext (black solid line) and their first four multipolar contributions: electric dipolar (red), magnetic dipolar (blue), electric quadrupolar (green) and magnetic quadrupolar (pink) are included. The grey area corresponds to the spectral range where dipolar terms dominate. In this region, Q ext presents two main peaks due to the excitation of either an electric dipolar (ED at λ =57 mm) or a magnetic dipolar (MD at λ =76 mm) resonance. Higher-order resonances are also observed (EQ: electric quadrupolar, MQ: magnetic quadrupolar). These resonant modes are consequence of the distribution of the electric field inside the particle (see inset which symbolically represents this distribution). ( b ) In the dipolar regime (grey area), the linear polarization degree at the right angle configuration, P L (90°), also identifies dipole resonances: the electric (positive values) and the magnetic (negative values). Experimental values of P L (90°) for the considered target ( a =9 mm and ε =16.5+0 i ) averaged over the different experimental configurations described in Fig. 1 (VC and +90° and –90° for the HC) are plotted as red dots. In addition, theoretical values of P L (90°) (see equation 5) are also included (black solid line) to show the excellent agreement between theory and experiment, even out of the dipolar regime ( λ <53 mm). Horizontal dot-dashed line corresponds to P L (90°)=0. Dotted vertical lines mark the incident wavelengths at which dipolar contributions, either electric or magnetic, cross each other ( a ). These wavelengths also coincide with those at which P L (90°)=0 ( b ). Full size image where θ is the scattering angle and α e and α m are the electric and magnetic polarizabilities of the sphere that can be written in terms of the Mie coefficients a 1 and b 1 as and ( k is the wave number , the induced dipoles in SI units are given by and and we use the convention ). As evidenced in equation 1, the interference between electric and magnetic dipoles leads to a number of interesting effects: the intensity in the backscattering direction ( θ =180°) is zero when a 1 = b 1 (first Kerker condition) with an overall pattern similar to that of a Huygens source. The zero backwards condition takes place at λ =84 mm ( a/λ ~0.11) as shown in Fig. 3a . Although the intensity cannot be exactly zero in the forward direction, the forward scattering ( θ= 0°) presents a minimum when Im( a 1 ) ~−Im( b 1 ) and | a 1 | 2 =| b 1 | 2 (refs 8 , 39 ). For ε ≈16.5+0 i this second Kerker condition takes place at λ =69 mm ( a/λ ~0.13). (Black dashed lines in Fig. 2 point to the incident wavelengths corresponding to Kerker conditions in the dipolar regime). It should be remarked that these conditions are the consequence of the coupling between the electric- and the magnetic-induced dipoles in the dielectric sphere (cf. equation 1). For incident wavelengths smaller than 52 mm, there are additional interference effects due to the interaction between dipolar and quadrupolar responses. As a classical analogue of Fano resonances [24] , [27] , [40] , [41] , [42] , [43] , constructive and destructive interference effects between sharp quadrupolar (or higher-order multipolar) resonances with broader dipolar modes lead to asymmetric Fano resonance profiles exhibiting sharp minima of the scattered intensities in the forward or backward directions [40] , [41] , [42] . As a complement to the main objective of our research, Supplementary Fig. S1 shows calculations exhibiting Kerker minima of both backward and forward scattered intensities, as well as those associated to some Fano resonances (see Methods). Linear polarization degree at 90° The highly asymmetric scattering is also reflected on the polarization of the scattered electromagnetic wave. A useful polarimetric parameter to see this is the degree of linear polarization, measured at a right-angle scattering configuration, P L (90°), defined in terms of the scattered intensities at 90° with respect to the incident wave direction for polarizations perpendicular (s) and parallel (p) to the plane of incidence, respectively. It is quite straightforward to show that the spectral evolution of this parameter involves a simple and accurate way to identify either electric or magnetic dipolar behaviours, as well as deviations from a purely dipolar response [37] , [38] . The predicted spectral evolution of P L (90°) computed from the full Mie series, is plotted in Fig. 3b (thick black line). In the dipolar region (grey area in Fig. 3b ) (see Methods), This parameter takes positive values for wavelengths for which an electric dipolar conduct is dominant, that is, when terms associated with a 1 dominate, while it is negative when the scattering behaviour is mainly governed by the dipolar magnetic term, associated with b 1 (ref. 38 ). In addition, the spectral evolution of P L (90°) reaches a maximum or a minimum when the electric or the magnetic dipolar resonances are excited, respectively. Figure 3b shows the experimental data for spectral evolution of P L (90°) (red filled dots). This result is the average of those obtained for the three considered experimental configurations (two for the horizontal configuration (HC):+90° and −90° and one for the vertical configuration (VC), see Fig. 1 ). The agreement is excellent with that predicted by the numerical simulations from Mie theory. The experimental spectral evolution of P L (90°) shows the positive maximum at short wavelengths ( λ ~57 mm), corresponding to a dominating dipolar electric behaviour, and a pronounced negative region, corresponding to a dominant dipolar magnetic mode ( λ ~76 mm). These results constitute the first demonstration with experimental data of the coexistence of electroinductive and magnetoinductive resonances for moderate high-refractive index dielectric particles. At shorter wavelengths the spectral evolution of P L (90°) becomes more complex due to the above-mentioned interference between dipolar and quadrupolar terms but still in good agreement with the full Mie theory. From a practical point of view, equation 2 is an interesting result as at the Kerker conditions, with |a 1 |=|b 1 |, P L (90°) is zero. In the dipolar regime, Kerker conditions can then be readily identified as zeros in the spectral evolution of P L (90°). In Fig. 3a and in the dipolar regime, the spectral evolution of P L (90 °) takes the value zero at two incident wavelengths, around 69.3 and 83.2 mm (vertical mark lines in Fig. 3 ). Far- and near-field scattering In Fig. 4a and b , we plot the far-field scattering patterns measured in the experiment (blue circles for the HC and red stars for the VC) for the considered dielectric sphere at these particular wavelengths, 84 and 69 mm, respectively, and for p incident polarization. Equivalent results are obtained for s incident polarization as predicted in ref. 8 . For illustrative purposes, we also plot in Fig. 4c and d , colour plots of the numerically calculated total near-field, in order to show how the scattered wave evolves from the near- to the far-field approximations and how they are correlated. Also, and for comparison purposes, simulated far-field scattering angular patterns for a spherical particle ( a =9 mm) and constitutive parameters: ε= 16.5+0 i , μ= 1, (ref. 1 ), are also shown in this figure (black line). The agreement between experiment and theory is excellent. For λ= 84 mm ( Fig. 4a ) the zero-backward scattering condition holds. This can be clearly observed in the angular distribution of the far-field scattered intensity where radiation in the backward hemisphere is strongly reduced, and it is almost suppressed in the backward direction. The electromagnetic scattering is almost inhibited throughout the whole backward hemisphere (180° <θ< 360°). In fact, 93% of the scattered energy in the plane is radiated into the forward hemisphere and only 7% remains in the backward one. Experimental results confirm this scattering behaviour at this wavelength. In this sense, and although an angle range of ~60° in HC and 15° in VC around the backward direction cannot be measured due to experimental constraints, it can be clearly concluded that the electric field is very weak in the surroundings of the backward direction and most of the scattered radiation energy is strongly concentrated in the forward hemisphere. 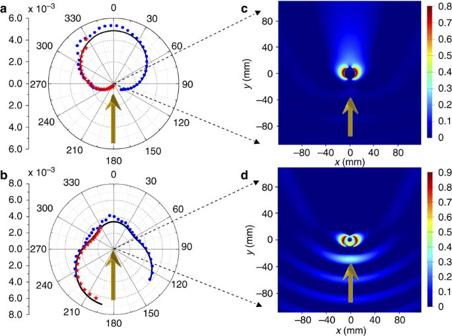Figure 4: Far- and near-field scattering patterns under Kerker conditions. (a,b) Experimental values (full circles/stars) of the scattered intensity of the considered target (sphere of radiusa=9 mm andε=16.5+0i,μ=1) when it is illuminated from below (see yellow arrows) by a p-polarized plane wave, which satisfies either the zero-backward condition (λ=84 mm) (a) or the minimum forward condition (λ=69 mm) (b). Both experimental configurations (seeFig. 1), HC (blue full circles) and VC (red stars), are considered. Theoretical results (black line) are also included for comparison purposes. (c,d) Calculated distribution of the total near-field intensity around the particle (logarithmic scale) for the same cases considered in (a) and (b), that is, when the incident wavelength satisfies either the zero-backward condition (c) or the minimum forward condition (d), respectively. Figure 4: Far- and near-field scattering patterns under Kerker conditions. ( a,b ) Experimental values (full circles/stars) of the scattered intensity of the considered target (sphere of radius a =9 mm and ε =16.5+0 i , μ =1) when it is illuminated from below (see yellow arrows) by a p-polarized plane wave, which satisfies either the zero-backward condition ( λ =84 mm) ( a ) or the minimum forward condition ( λ =69 mm) ( b ). Both experimental configurations (see Fig. 1 ), HC (blue full circles) and VC (red stars), are considered. Theoretical results (black line) are also included for comparison purposes. ( c,d ) Calculated distribution of the total near-field intensity around the particle (logarithmic scale) for the same cases considered in ( a ) and ( b ), that is, when the incident wavelength satisfies either the zero-backward condition ( c ) or the minimum forward condition ( d ), respectively. Full size image At λ= 69 mm, P L (90°)=0, and the zero-forward scattering condition holds ( Fig. 4b ). In contrast with the previous case, an exact zero-forward scattering cannot be obtained due to energy conservation constraints [15] , [39] , [44] . However, most of the scattered energy is located in the backward hemisphere with a 73% versus a 27% in the forward hemisphere. This spatial distribution of the scattered radiation energy also confirms this particular behaviour with an excellent agreement between experiment and numerical predictions (black line). These experimental results clearly confirm the analysis made by Kerker et al . [8] We have confirmed unambiguously by experiments in the microwave range ( v ~3–9 GHz → λ ~33–100 mm) that subwavelength spherical particles of moderatly high-refractive index (≈3–4) are able to scatter light according to the theoretical predictions made by Kerker et al . [8] over thirty years ago. The spectral behaviour of a useful polarimetric parameter, the degree of linear polarization measured at a right-angle scattering configuration, P L (90°), has helped to corroborate those predictions. It is quite straightforward to show that this parameter involves a simple and accurate way to identify clearly either electric or magnetic dipolar behaviours, as well as deviations from a purely dipolar response. Also, P L (90°) has permitted to locate the spectral position of the Kerker frequencies ( P L (90°)=0) where destructive interference between the scattered fields by the induced electric and magnetic dipoles in the particle produces minima in the forward and backward scattering directions. The interesting consequences of the coherent effects between the scattered fields generated by the induced electric and magnetic dipoles in a single dielectric particle, like zero-backward and almost zero-forward scattering should be the basis of sophisticated antenna arrangements in the microwave range to achieve directionality and other interesting scattering effects ‘à la carte’. The rescaling property of the analysed scattering problem makes these results immediately extendable to other spatial ranges (micro-nano) and consequently to other spectral ranges (near-infrared to visible). This can open up new technological challenges, for instance in the optical region. Theoretical methods The angular distribution of the scattered electromagnetic wave by a spherical particle of radius a, is usually described by means of its scattered irradiance (normalized to the incident irradiance). Their components parallel (p) and perpendicular (s) to the scattering plane in a given direction θ with respect to the incident beam direction can be expressed, respectively, as follows [1] a n and b n being the Mie coefficients associated, respectively, to the electric and magnetic n-polar contribution and τ n and π n being ‘ θ -dependent functions’ [1] . The scattered electromagnetic radiation contains information about the scatterer not only in how its energy is redistributed in space but also in how is its polarization. In our case, we have chosen to study the spectral behaviour of the linear polarization degree measured at the right-angle scattering configuration, P L (90°), defined as For subwavelength scatterers, the value of the scattered electromagnetic field can be well approximated by using only the first terms of the multipolar expansion. For very small particles ( a/λ <<1), both the electric and the magnetic scattered fields can be properly described by using the first four Mie terms. These correspond to the dipolar and quadrupolar contributions, both electric and magnetic, which are associated to the Mie coefficients a 1 , a 2 , b 1 and b 2 , respectively. Under this approximation, the polarized components of the scattered irradiance are if the incident light is polarized parallel (s) to the scattering plane, and if the incident light is polarized perpendicular (p) to the scattering plane. From the two polarized components of the scattered intensity, (equations 6, 7), the linear polarization degree at the right-angle scattering configuration, P L (90°), can be expressed as However, when dipolar contributions electric and/or magnetic dominate, only the Mie coefficients of first order, a 1 and b 1 , are not negligible and equation 8 can be approximated by It can be observed that when an electric dipolar behaviour dominates ( a 1 tends to dominate), P L (90°) acquires positive values, while if P L (90°) is negative, the dominant behaviour is magnetic ( b 1 gets larger values than a 1 ) [38] . When | a 1 |=| b 1 |, P L (90°)=0 and Kerker conditions hold [8] . Two interesting scattering directions are the forward ( θ= 0°) and the backward ( θ= 180°) ones. For these, the scattered irradiance for the considered target, under a dipole-quadrupole expansion approximation, can be written as Equations 10, valid for both s and p polarizations, show that coherent effects occur between both electric and magnetic dipoles, as well as between dipolar and quadrupolar modes, producing interesting phenomena in the spectral behaviour of the scattered intensity in these directions. In particular, when quadrupolar and higher-order multipoles are negligible, the electric and the magnetic dipolar contributions interfere, either constructively or destructively, producing minima in either the backward or the forward scattered intensity at certain incident frequencies [26] . These Kerker frequencies are marked by arrows in Supplementary Fig. S1 for a dielectric sphere with a =9 mm and ε =16.5+0 i . Forward scattering (upper part of Supplementary Fig. S1a ) reaches two minima around 4.3 and 6.3 GHz, respectively (second Kerker condition), when the real parts of a 1 and b 1 match and their imaginary parts are equal but with different sign ( Supplementary Fig. S1b ). In a similar way, a drop appears in backward scattering (bottom part of Supplementary Fig. S1a ) at 3.6 GHz corresponding to the matching of the real and imaginary parts of Mie coefficients a 1 and b 1 (first Kerker condition) ( Supplementary Fig. S1b ). It is important to point out that while the optical theorem imposes a theoretical minimum value for the forward scattered intensity, the minimum of backscattering is limited by the negligible contribution of quadrupolar modes at low frequencies and the experimental resolution. Another Kerker minimum of the backscattered intensity, mainly contributed by the interference of a 1 and b 1 with a minor contribution from Re( a 2 ) and Re( b 2 ), can be observed at 8 GHz (bottom part of Supplementary Fig. S1a ). For frequencies higher than 5.5 GHz (incident wavelengths shorter than 54 mm), there are additional interference effects due to the interaction between dipolar and quadrupolar responses. Constructive and destructive interference effects between sharp quadrupolar (or higher-order multipolar) resonances with broader dipolar modes lead to asymmetric Fano resonance profiles exhibiting minima of the scattered intensities in the forward or backward directions [40] , [41] , [42] . The minima of the intensity in the forward direction at 5.7 GHz (red-shifted with respect to the magnetic quadrupolar resonance at 5.8 GHz) and at 6.2 GHz in the backward direction, can be associated to the quadrupolar magnetic Fano resonance arising from the interference of b 1 and b 2 with a minor contribution from the electrical terms. Notice that the constructive or destructive interference depends on the signs of the imaginary part of the Mie coefficients [40] ( Supplementary Fig. S1b ). For example, the Fano shape of the electrical quadrupolar resonance (at 7.2 GHz) is similar to the magnetic quadrupole but with the minima blue-shifted in the forward direction and red-shifted in backscattering (see the sharp backwards minimum at 7 GHz). The spectrum below 7.4 GHz (the frequency of the magnetic octupolar resonance) is perfectly well described by only dipolar and quadrupolar modes (equation 10). The analysis of the spectrum at shorter wavelengths becomes more complex due to partial contributions from several Mie coefficients. Experimental methods Our experiments have been performed in an anechoic chamber at the Centre Commun de Ressources Microondes (Institute Fresnel, Marseille, France), originally designed for SER/diffraction [45] , [46] and antenna characterization [47] . This facility was successfully used for carrying out microwave analogue to light scattering measurements on various kinds of complex particles [48] . The experimental setup in Fig. 1 allows measuring scattered fields (both in magnitude and phase) on a spherical surface of nearly 4 m in diameter, surrounding the scattering target under test. In the present work, the measurements have been much more challenging as the target is a single sphere of 9 mm in radius, that is, a/λ is between 0.1 and 0.25 at our working frequencies. It is made of a material (ECCOSTOCK-HIK from Emerson and Cuming. http://www.eccosorb.com/ ) with a permittivity similar to that of some semiconductor materials (Si, Ge), with almost no dispersion in the frequency range of interest, and very low losses (the dissipation factor is given to be <0.002 in the 1 to 10 GHz range). In order to determine, as accurately as possible, the permittivity of the material at the working frequencies, some extra measurements have been done with a sphere of 12 mm in radius made of the same material. Thus, assuming a null imaginary part, by comparing the measured scattered field of this sphere to Mie calculations, we have estimated the permittivity of the material to be ε ≈ 16.5+0 i (see Supplementary Methods ). This value has been selected in all the computations and analysis made in this research. The scattering target is positioned at the centre of the sphere of measurement, on a polystyrene mast almost transparent in the frequency range of study. The antennas are broadband ridged horns (ARA DRG118), emitting linearly polarized microwaves, either with s (perpendicular to the scattering plane) or p (parallel to the scattering plane) polarizations (see Fig. 1 ), which are conveniently obtained by a rotation of the antennas. All measurements presented here have been made in configurations such that the transmitter, the target and the receiver are kept in either the horizontal or the vertical planes (HC and VC, respectively, in Fig. 1 ). There are two main advantages to perform the measurements in those two configurations. Indeed, the first advantage is that the environment of the source is not the same in the two cases, thus the parasitic signals are different. This also allows to determine the linear polarization degree at a right-angle configuration ( P L (90°)) in three different experimental conditions (two for the HC:+90° and –90°; one for the VC). The second advantage is that one can obtain a more complete measurement of the scattering pattern from the sphere because of the different angular possibilities. In fact, due to the low a / λ ratio, the scattered intensity is really small and very sensitive to any perturbation from parasitic echoes, stray signals, drift problems or even due to the non-linearity of the receiver. Furthermore, the problems are amplified by the fact that, to extract the field scattered from the measurements, we need to acquire two complex fields: that is, the total field from the scattering measurements, (which contain both the forward non-scattered part of the incident field plus that scattered by the sphere), and the field detected without the presence of the sphere, (namely, the incident field). Then, we a posteriori subtract that incident field from the total one to obtain the scattered field. Owing to the difficulty of those scattering measurements, in order to obtain reliable results, a calibration procedure and two types of post-processing of the data have been used, the first one compensates for the drift phenomenon, while the second one consists of a time gating filtering to remove as much as possible the stray signals [49] (see Supplementary Figs S2 to S7 and Supplementary Methods for specific details). How to cite this article: Geffrin, J.M. et al . Magnetic and electric coherence in forward- and back-scattered electromagnetic waves by a single dielectric subwavelength sphere. Nat. Commun. 3:1171 doi: 10.1038/ncomms2167 (2012).